Ultrafast changes in lattice symmetry probed by coherent phonons The electronic and structural properties of a material are strongly determined by its symmetry. Changing the symmetry via a photoinduced phase transition offers new ways to manipulate material properties on ultrafast timescales. However, to identify when and how fast these phase transitions occur, methods that can probe the symmetry change in the time domain are required. Here we show that a time-dependent change in the coherent phonon spectrum can probe a change in symmetry of the lattice potential, thus providing an all-optical probe of structural transitions. We examine the photoinduced structural phase transition in VO 2 and show that, above the phase transition threshold, photoexcitation completely changes the lattice potential on an ultrafast timescale. The loss of the equilibrium-phase phonon modes occurs promptly, indicating a non-thermal pathway for the photoinduced phase transition, where a strong perturbation to the lattice potential changes its symmetry before ionic rearrangement has occurred. The ultrafast control of a material's properties via non-equilibrium states is a new method to manipulate and control the structural [1] , magnetic [2] and electrical [3] properties of materials that may not be accessible under equilibrium conditions. The timescale on which one phase is lost and a new phase emerges is of fundamental interest for understanding how these transitions occur as well as being important for potential applications. However, as these transitions occur via non-equilibrium processes [4] , the parameters that define a phase and mark when a transition occurs are difficult to identify. In a structural transition, for example, the positions of ions within a crystal are determined by the interactions between the ions and electrons, with the ions residing at minima of the resulting lattice potential energy surface. The lattice potential also determines, through its curvature, the phonon spectrum of the solid, that is, the response to external perturbations. In most cases, when a solid undergoes a structural phase transition, the symmetry of the lattice potential changes. This modifies both the ionic positions and the phonon spectrum. In equilibrium, these changes are concomitant; however, out of equilibrium the lattice potential may change before the ions have reached their new positions. In such a situation, the photoinduced change in the potential defines the onset of the phase transition. A material's structure can be measured by elastic X-ray or electron diffraction, which maps ionic positions into specific Bragg peaks. Changes in ionic positions are observed by changes to these peaks and, by extending this technique to the time domain, dynamical phase transitions can be clearly identified [5] , [6] , [7] , [8] . However, the equivalent analysis of the time-resolved changes in the phonon spectrum during a time-dependent phase transition has received less attention. Yet the evolution of the phonon spectrum may clarify the description of phase transitions, as changes in the potential are responsible for the forces that drive the transition into the new phase. Phonon spectra can be measured via Raman scattering, which measures the Raman active modes at the Γ-point of the Brillouin zone. This technique can be extended into the time domain to reveal transient symmetry changes [9] , but the time resolution of these experiments is typically low. To overcome this limitation, coherent phonon generation can be used. In an absorbing material, laser light redistributes charge within the solid. This perturbs the lattice potential and produces a force on the ions. The response of ions to the force is determined by the normal modes of the potential, which are expressible as a superposition of phonon modes [10] . If the force generated is fast compared with the period of the phonon, then coherent motions of the lattice, or coherent phonons, are induced. This motion can be tracked in the time domain by measuring the effects of the coherent phonons on the transient reflectivity of a material and has been used extensively as a probe to study the lattice in near-equilibrium conditions in the vicinity of phase transitions [11] , as well as to look at phonon softening [12] , [13] , [14] and hardening [15] when the system is strongly driven. Phonon softening or hardening results from a change in the curvature [16] , [17] of the lattice potential, but not from a change in the symmetry of the potential. When the symmetry changes, the number of modes typically changes, which may occur when a soft phonon mode tends to zero frequency for a second-order phase transition [14] or may be step-like for a first-order phase transition. In this article, we demonstrate this principle using the photoinduced phase transition in VO 2 . A prompt change in the number of modes is observed at high excitation densities, providing an unambiguous marker for the structural phase transition on the ultrafast timescale. These measurements clarify the nature of the photoinduced phase transition mechanism; the pump laser induces, via strong electronic excitations, a prompt change of the symmetry of the lattice potential, which acts as the driving force for the non-thermal transition, as evidenced by the ultrafast change in the coherent phonon spectrum. These results indicate new ways in which ultrafast structural transitions can be measured through optical probes. Phonons during the photoinduced phase transition in VO 2 At room temperature, VO 2 is a monoclinic M 1 -phase insulator with P2 1/c space group, consisting of four vanadium ions per unit cell. On heating above T c =343 K, VO 2 becomes metallic and undergoes a first-order structural phase transition to a rutile R-phase with the space group P4 2/mnm , with only two vanadium ions per unit cell. The increased symmetry reduces the number of Raman active phonon modes from 18 in the M 1 phase to 4 in the R-phase, without any significant mode softening near the transition temperature [18] . The same structural transition has been induced on the ultrafast timescale by exciting M 1 -phase VO 2 at room temperature with an intense 800 nm pump laser, using a pump fluence greater than F th ~7 mJ cm −2 , and observed by femtosecond X-ray [6] , [19] and electron diffraction [7] , as well as through changes in the optical [20] , [21] and electrical [22] , [23] properties. These experiments show that the complete transformation to the R-phase, after some initial fast dynamics, is a slow process, taking hundreds of picoseconds to complete. However, measurements of the rising edge of the optical transient suggested that the phase transition occurred on a timescale limited by the phonon modes of M 1 -phase VO 2 (ref. 21 ). 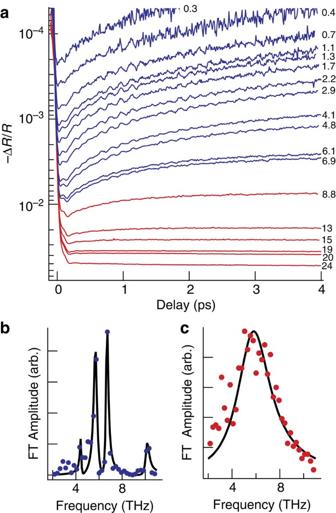Figure 1: Dynamics of the reflectivity at 800 nm across the photoinduced phase transition. (a) Transient reflectivity at 800 nm as a function of pump fluence. The numbers to the right of each transient indicate the pump fluence measured in mJ cm−2. Blue lines correspond to transients below the 7 mJ cm−2threshold, red lines above. Fourier transforms (FT) of the transient reflectivity after subtracting a fitted background (seeMethods) for (b) below threshold (1.7 mJ cm−2) and (c) above (24 mJ cm−2). Below threshold the four lowest Raman active modes are clearly observed (solid line indicates the best fit to four Lorentzian oscillators). Above threshold, all M1phonons are lost and a single broad feature is observed. Figure 1a shows the transient reflectivity of VO 2 measured using 800 nm, 40 fs pump and probe laser pulses for multiple pump fluences at room temperature. Several clear features can be observed. First, there is a large transient that decays back to the initial value with a time constant that depends on fluence. For pump fluences below threshold, oscillations also modulate the transient reflectivity, which are the result of the excitation of coherent M 1 -phase phonons by the pump pulse. Fig. 1b shows a Fourier transform of these oscillations, taken from −300 fs to 4 ps, after subtracting the non-oscillating transient by fitting a two-component exponential decay (see Methods ). Four distinct peaks are observed in the spectrum at 4.4, 5.7, 6.7 and 10.2 THz (147, 191, 224 and 340 cm −1 ). These frequencies correspond to the four strongest Raman active phonon modes of the M 1 phase that can be coherently excited by our pulse and are in good agreement with those reported in the literature [18] . Figure 1: Dynamics of the reflectivity at 800 nm across the photoinduced phase transition. ( a ) Transient reflectivity at 800 nm as a function of pump fluence. The numbers to the right of each transient indicate the pump fluence measured in mJ cm −2 . Blue lines correspond to transients below the 7 mJ cm −2 threshold, red lines above. Fourier transforms (FT) of the transient reflectivity after subtracting a fitted background (see Methods ) for ( b ) below threshold (1.7 mJ cm −2 ) and ( c ) above (24 mJ cm −2 ). Below threshold the four lowest Raman active modes are clearly observed (solid line indicates the best fit to four Lorentzian oscillators). Above threshold, all M 1 phonons are lost and a single broad feature is observed. Full size image On increasing the fluence, the amplitudes of these modes increase up to F th , at which point they are reduced and disappear, leaving the decaying transient to dominate the dynamics. This is indicated in Fig. 1c , which shows the Fourier transform of the signal when excited well above the phase transition threshold, after background subtraction. In this case, the signal consists of a single broad feature, and the normal modes of the monoclinic phase cannot be identified. Broadband spectroscopy The complete loss of the four M 1 -phase phonons suggests a change in the symmetry of the lattice potential. However, due to the large background it is difficult to determine whether the loss of the phonon modes is instantaneous or due to a dephasing mechanism. To clarify this, we performed broadband probing of the phase transition. 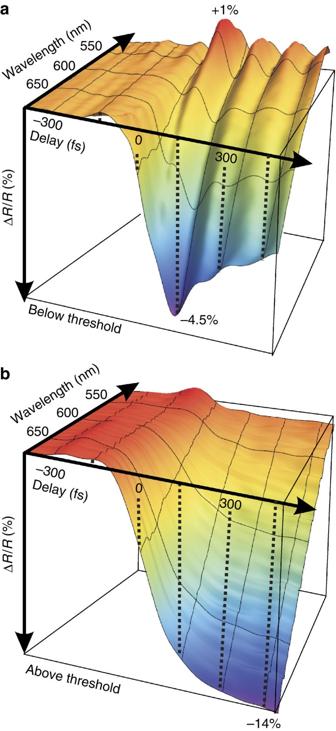Figure 2: Broadband transient spectroscopy of the photoinduced phase transition. Transient reflectivity as a function of probe wavelength and delay, (a) below and (b) above the photoinduced phase transition threshold. Below threshold, signals at longer wavelengths are dominated by a large negative transient with the oscillations dominating the signal at shorter wavelengths. Above threshold, no oscillations are observed, showing that the phonon modes are lost over the entire visible spectrum. Figure 2a shows 800-nm pump-induced changes in the room temperature reflectivity from 520 to 700 nm for below threshold excitation. At all wavelengths coherent oscillations are observed, yet the decaying background is only prominent at longer wavelengths and becomes significantly smaller than the phonon modulation at shorter wavelengths. In line with the observations made with 800-nm probe pulses, the phonons disappear across the whole probed spectrum above the phase transition threshold ( Fig. 2b ), demonstrating that the loss of phonon modes is not an optical probe–related artefact. These transient changes in reflectivity are also consistent with the temperature-driven change in reflectivity observed in thin films over the probed region, which show a smaller decrease at shorter wavelengths and a large decrease near 700 nm (ref. 24 ). Figure 2: Broadband transient spectroscopy of the photoinduced phase transition. Transient reflectivity as a function of probe wavelength and delay, ( a ) below and ( b ) above the photoinduced phase transition threshold. Below threshold, signals at longer wavelengths are dominated by a large negative transient with the oscillations dominating the signal at shorter wavelengths. Above threshold, no oscillations are observed, showing that the phonon modes are lost over the entire visible spectrum. 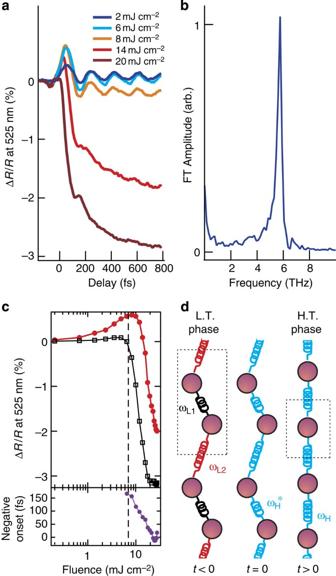Figure 3: Evolution of the phonon modes during the photoinduced phase transition. (a) The evolution of the reflectivity at a probe wavelength of 525 nm for various fluences. (b) The Fourier transform (FT) of the 2 mJ cm−2transient without background subtraction. (c) Fluence dependence of peak signal measured at 60 fs (red circles) and the background level measured at 4 ps (black open squares), demonstrating that the phonon amplitude increases until the transition threshold (dashed line at 7 mJ cm−2) at which point the negative transient dominates. Also plotted (purple circles) is the time after excitation at which a negative change in reflectivity is observed (defined as when the reflectivity change decreases below −0.1%). At the highest fluences the onset of the negative transient is limited by the pulse duration. (d) Simplified schematic of the phase transition in VO2. Low-temperature (L.T.) and high-temperature (H.T.) vanadium positions are shown, which are also the positions before (t<0) and after (t>0) excitation. The low and high temperature phases can be characterized by a different set of spring constants ωx, which are promptly changed after excitation. Att=0, the lattice potential is changed before significant atomic motion. Dashed boxes represent the unit cells. Full size image Figure 3a shows the transient reflectivity of p -polarized 525-nm light after spectral filtering the broadband probe to 5-nm bandwidth, at several pump fluences. At this wavelength, and at low fluences, the transient reflectivity shows a small positive background and is particularly strongly modified by the 5.7-THz phonon, as shown by the Fourier transform of the raw data in Fig. 3b . On increasing the pump fluence, the positive phonon amplitude increases until the phase transition threshold is reached. At this point the phonon amplitude decreases to zero, and a negative transient appears. This is highlighted in Fig. 3c , which plots the change in reflectivity at the peak of the phonon amplitude as well as the reflectivity change of the non-oscillatory signal at 4 ps delay. Also shown in Fig. 3c is the time delay at which a negative reflectivity is first observed (defined as the delay when the reflectivity decrease is >0.1%), which is indicative of the phase transition. This occurs earlier with increasing fluence and, at the highest fluences, occurs during the laser pulse. This, together with the loss of coherent M 1 -phase phonons, indicates that the symmetry of the lattice potential is changed during the excitation process. Figure 3: Evolution of the phonon modes during the photoinduced phase transition. ( a ) The evolution of the reflectivity at a probe wavelength of 525 nm for various fluences. ( b ) The Fourier transform (FT) of the 2 mJ cm −2 transient without background subtraction. ( c ) Fluence dependence of peak signal measured at 60 fs (red circles) and the background level measured at 4 ps (black open squares), demonstrating that the phonon amplitude increases until the transition threshold (dashed line at 7 mJ cm −2 ) at which point the negative transient dominates. Also plotted (purple circles) is the time after excitation at which a negative change in reflectivity is observed (defined as when the reflectivity change decreases below −0.1%). At the highest fluences the onset of the negative transient is limited by the pulse duration. ( d ) Simplified schematic of the phase transition in VO 2 . Low-temperature (L.T.) and high-temperature (H.T.) vanadium positions are shown, which are also the positions before ( t <0) and after ( t >0) excitation. The low and high temperature phases can be characterized by a different set of spring constants ω x , which are promptly changed after excitation. At t =0, the lattice potential is changed before significant atomic motion. Dashed boxes represent the unit cells. Full size image Such an ultrafast change in the lattice potential is shown in the schematic of Fig. 3d . The initial low-temperature phase of VO 2 is a distorted chain of vanadium ions. This distortion produces multiple optical phonons, simply represented here as ω L1 , as well as acoustic phonons, ω L2 . Photoexcitation brings the system to the high temperature rutile phase, with a reduced unit cell and a reduced phonon spectrum, represented by a single phonon ω H , with no Raman active phonons involving vanadium ionic motions. The ultrafast change in the lattice potential is indicated in the middle schematic of Fig. 3d , where the laser pulse has changed the lattice potential, and thus the phonon spectrum, before the structure has had significant time to respond. As a result, a displacive excitation is no longer capable of producing coherent phonons. Probing the excited state At this point, it should be noted that the transient dynamics shown in Figs 1 and 2 result from multiple processes in addition to coherent phonons, such as the electronic response and coherent interactions between laser beams. These may give rise to additional features (for example, the kink observed at 180 fs in the 20 mJ cm −2 trace in Fig. 3a ), which may not be easily distinguished from coherent phonons. Therefore, to verify that the symmetry change occurs during the excitation process, we perform a pump-probe experiment on the excited state of the system below and above the phase transition threshold. Such a technique has been previously used to demonstrate the effects of damping of soft modes [25] , [26] , [27] . 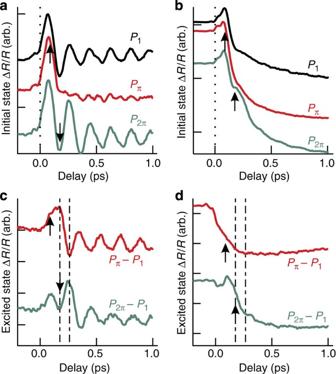Figure 4: Probing the response of the excited state. Pump–pump-probe measurements (a) below threshold and (b) above. Traces labelledP1correspond to the transient reflectivity generated by a single pump pulse. Traces labelledPπandP2πcorrespond to a double-pulse excitation when the pump–pump delay is set to be out of phase,Pπ, or in-phase,P2π, with the 5.7-THz phonon mode. The arrows indicate the arrival time of the second pump pulse. Panelscanddcorrespond to the transient response of the excited state below and above threshold, respectively, obtained by subtracting the single-pulse transient reflectivity from the double-pulse transient reflectivity. Dashed lines correspond to the points separated by half of the 5.7-THz phonon period, which are anticorrelated below threshold and exhibit no correlation above threshold. Figure 4 shows the results at a probe wavelength of 525 nm. Here the first pulse P 1 excites the system and after a time τ 12 a second pump P 2 excites the transient state. The probe pulse then measures the combined response, P x ( t )= P 1 ( t )+ P 2 ( t −2π x / ω ), where ω is the frequency of the phonon mode. Transients are shown for single pump excitation, P 1 , and for when the pump–pump delay is set to be half a period, P π (88 fs), and a full period, P 2π (176 fs), of the 5.7-THz phonon. In Fig. 4a , the fluence of P 1 is below threshold, while it is above it in Fig. 4b . The effect of P 2 on the time-dependent reflectivity of the excited state can be extracted by subtracting P 1 from the measured combined signal, that is, P x − P 1 , which is shown in Fig. 4c and d for below and above threshold, respectively. Figure 4: Probing the response of the excited state. Pump–pump-probe measurements ( a ) below threshold and ( b ) above. Traces labelled P 1 correspond to the transient reflectivity generated by a single pump pulse. Traces labelled P π and P 2π correspond to a double-pulse excitation when the pump–pump delay is set to be out of phase, P π , or in-phase, P 2π , with the 5.7-THz phonon mode. The arrows indicate the arrival time of the second pump pulse. Panels c and d correspond to the transient response of the excited state below and above threshold, respectively, obtained by subtracting the single-pulse transient reflectivity from the double-pulse transient reflectivity. Dashed lines correspond to the points separated by half of the 5.7-THz phonon period, which are anticorrelated below threshold and exhibit no correlation above threshold. Full size image In the low fluence regime ( P 1 =4.4 mJ cm −2 , P 2 =1.7 mJ cm −2 , P 1 + P 2 < F th ), the phonon amplitude is switched on and off by the presence of P 2 , as P 2 creates phonons that are either in-phase ( P 2π ) or out ( P π ) of phase with those generated by P 1 . This can be seen by the values of the transient reflectivity changes at the dashed lines in Fig. 4c , which are separated by half a phonon period, and show a π-phase shift. In this case, the combined fluence is below the phase transition threshold and the phonon mode does not exhibit a significant red-shift in frequency, suggesting that this mode does not significantly soften before the phase transition, as observed in static Raman scattering [18] . Control over the amplitude of the phonon mode is only possible because the symmetry of the lattice potential, and thus the restoring forces, does not change after excitation with P 1 . However, if P 1 is above the threshold and changes the lattice potential on an ultrafast timescale, it should not be possible for P 2 to excite coherent phonons that are characteristic of the M 1 phase. This is observed in Fig. 4c , where P 1 is above the phase transition threshold (10 mJ cm −2 ) and P 2 is below (3 mJ cm −2 ). As shown in Fig. 4d , no correlated response, in-phase or out-of-phase with P 1 , is observed in the excited transients, demonstrating that the phonon modes have been lost and no coherent motion can be induced in the excited state of the system. Instead, the second pulse generates an additional large negative transient. The same result was observed when probing at 800 nm, but with a much larger background transient. This shows that the observed peak at ~180 fs in the 20 mJ cm −2 transient of Fig. 3c is not the result of a damped oscillation of the M 1 phase. Such a feature may correspond to plasmons [28] or even squeezed phonons [29] that cannot be induced by the weaker second pulse. However, at these high fluences, the intensity in the wings of P 1 , which would otherwise be negligible, may become significant and could also affect the optical signal. The loss of all the M 1 modes after the 40-fs pump pulse indicates that the entire potential symmetry has changed on an ultrafast timescale. This occurs when a sufficient number of electrons are excited so that their perturbation to the lattice potential becomes large enough to modify the symmetry, subsequently driving the system, non-thermally, into the R-phase. The interpretation of the ultrafast structural phase transition in VO 2 that results from these measurements differs from the previously proposed mechanism, in which the timescale was said to be dictated by the phonon period of the monoclinic phase [6] . On the contrary, at high fluences we observe a complete loss of the coherent motion associated with the monoclinic phase and a drastic change in the response of the excited state, demonstrating a change in symmetry of the lattice potential that is promptly driven by the laser pulse. This analysis brings the ultrafast phase transition mechanism of VO 2 into agreement with other Peierls-distorted materials such as bismuth, where the system melts on a subphonon-period timescale [8] . However, unlike bismuth, the transition in VO 2 involves complex changes in multiple phonons and results in a final state that is also an ordered solid. It should be emphasized that the establishment of the R-phase with long-range order is a slow process, occurring over tens of picoseconds [7] , that takes much longer than the observed loss in phonon modes [6] , [7] , [19] . The state of VO 2 immediately after photoexcitation is far from equilibrium, and the lattice potential is likely to continue to evolve to that of the R-phase during the thermalization process [30] , [31] . On these timescales, the evolution of the lattice and the electronic structure may not be concurrent, but may be accessible optically through the analysis of the broadband dielectric function [32] , [33] . The analysis presented here is general and can be applied to any ultrafast structural phase transition that changes the symmetry of the Raman tensor, providing an unambiguous ultrafast optical marker for all-optical probing of changes in the lattice potential and its symmetry. In addition, measuring the formation time of the new high-symmetry-phase phonon modes that result from the phase transition will provide new information on the establishment of long-range order in the system. Thus, the study of coherent phonons across photoinduced phase transitions is an ideal complement to time-resolved X-ray measurements. As coherent phonons result from prompt changes in the lattice potential, which generate the forces experienced by the ions, they can provide new insight into the mechanisms that drive non-equilibrium phase transitions compared with probes of ionic positions. Samples Experiments were performed on a 200-nm thin film of VO 2 grown on n -doped silicon via pulsed laser deposition [34] . The thermal phase transition was observed at 343 K on heating, and the thermal hysteresis was 10 K wide. Transient reflectivity The transient reflectivity was measured at a 50° angle of incidence and performed at room temperature. Measurements of 800 nm pump and 800 nm probe were performed at a laser repetition rate of 150 kHz and measured with a lock-in amplifier. Experiments of 800 nm pump white-light probe were performed at 100 kHz repetition rate. The duration of the 800-nm pulse was <40 fs. The white-light pulses were compressed and characterized, as described in ref. 35 , to ~11 fs duration. The spectrally resolved transient reflectivity was measured directly on a spectrometer, allowing the entire spectrum to be obtained at each time delay. Measurements at 525 nm were performed by spectrally filtering the broadband white-light pulse to 5-nm bandwidth after reflecting from the VO 2 sample and measured on a diode with a lock-in amplifier. Fourier transforms of 800 nm data The Fourier transforms shown in Figs 1b and c were performed after subtracting the non-oscillating transient by fitting a background function to the data show in Fig. 1a of the form Δ R ( t )/ R =(erf( t / τ p )+1)×( A 1 exp(− t / τ 1 )+ A 2 exp(− t / τ 2 )), where erf( t / τ p ) is the error function and represents the rising edge of the signal, which is dictated by the laser pulse duration τ p , which is independent of the pump power, and A i and τ i ( i =1, 2) are the fit parameters that represent the amplitude and recovery rate of the dynamics, respectively. How to cite this article: Wall, S. et al . Ultrafast changes in lattice symmetry probed by coherent phonons. Nat. Commun. 3:721 doi: 10.1038/ncomms1719 (2012).